Electrochemical tuning of layered lithium transition metal oxides for improvement of oxygen evolution reaction Searching for low-cost and efficient catalysts for the oxygen evolution reaction has been actively pursued owing to its importance in clean energy generation and storage. While developing new catalysts is important, tuning the electronic structure of existing catalysts over a wide electrochemical potential range can also offer a new direction. Here we demonstrate a method for electrochemical lithium tuning of catalytic materials in organic electrolyte for subsequent enhancement of the catalytic activity in aqueous solution. By continuously extracting lithium ions out of LiCoO 2 , a popular cathode material in lithium ion batteries, to Li 0.5 CoO 2 in organic electrolyte, the catalytic activity is significantly improved. This enhancement is ascribed to the unique electronic structure after the delithiation process. The general efficacy of this methodology is demonstrated in several mixed metal oxides with similar improvements. The electrochemically delithiated LiCo 0.33 Ni 0.33 Fe 0.33 O 2 exhibits a notable performance, better than the benchmark iridium/carbon catalyst. Water splitting with the assistance of either electricity or sunlight is able to provide a sustainable source of hydrogen, which is regarded as a clean energy carrier for powering fuel cells and reducing CO 2 to fuels [1] , [2] , [3] , [4] , [5] , [6] . One of the critical steps is oxygen evolution reaction (OER), which can be expressed as equation (1) in base solution. However, this half reaction proceeds via a multistep four-electron oxidation, and thus is kinetically sluggish [7] . An effective electrocatalyst is needed to accelerate the reaction, reduce the overpotential to obtain a current density of 10 mA cm −2 for matching with sunlight flux and thereby enhance the energy conversion efficiency. For this reason, a number of catalysts have been identified with low OER overpotentials [8] , [9] , [10] , [11] . The most active OER catalysts are IrO 2 or RuO 2 (refs 12 , 13 ), but the scarcity and high cost of these precious metals limit their large-scale application. Co-based compounds (for example, cobalt phosphate (CoPi) [14] , Co-containing perovskites [15] and Co 3 O 4 (ref. 16 )) have been proven to be competitive catalysts to precious metal oxides as a result of their good OER activity, easy accessibility and abundance. Theoretical simulations and experimental evidence have shown that the OER activity is highly related to the electronic structure of the Co atom, including oxidation state, e g filling and O p-band center [15] , [17] , [18] , [19] . While the search for materials with new chemical compositions continues to be an interesting direction to pursue, another approach is to develop methods to tune the electronic structure of existing materials in a wide dynamic range to optimize their catalytic activities. In the past two decades, electrochemical insertion and extraction of lithium ions in organic electrolyte have been studied in rechargeable battery materials, such as LiCoO 2 , a Co-based layered material [20] . Accompanied with this process, the control of atomic ratios and the tuning of the electronic structure have also been developed [21] , [22] . We hypothesize that such a continuous electronic structure tuning of oxide materials over a large potential range provides the opportunity for improving OER catalytic activity. Indeed, our recent study has demonstrated that the electronic structure of MoS 2 vertically layered nanofilm can be tuned by the electrochemical lithium intercalation process in organic electrolyte, which results in significant improvement of the subsequent hydrogen evolution reaction (HER) activity in aqueous solution [23] . The success with HER motivates us to use lithium electrochemical tuning for OER. Here we present our results on improving OER activities in LiCoO 2 and other Co-based compounds. We first study LiCoO 2 since it is one of the most well-known cathode materials used in current lithium ion batteries. We show that the delithiated LiCoO 2 (denoted as De-LiCoO 2 ), that is, the product obtained by charging LiCoO 2 to a high potential, exhibits remarkably enhanced OER activity compared to that of pristine LiCoO 2 . To demonstrate the general efficacy of this electrochemical tuning methodology for OER, we further examine a series of Co-based alloy oxides including LiCo 0.5 Ni 0.5 O 2 , LiCo 0.5 Fe 0.5 O 2 , LiCo 0.33 Ni 0.33 Fe 0.33 O 2 and LiCo 0.33 Ni 0.33 Mn 0.33 O 2, and find that the OER activities of delithiated products are all improved significantly. Particularly, the delithiated LiCo 0.33 Ni 0.33 Fe 0.33 O 2 shows the best performance with onset potentials of ~1.47 V versus reversible hydrogen electrode (RHE) and ~1.525 V at 10 mA cm −2 , even better than commercial Ir/C catalyst and comparable to the best OER catalysts reported so far [8] , [14] , [15] . Synthesis and OER performance of De-LiCoO 2 A porous polymer precursor procedure previously developed in our group was employed for synthesizing LiCoO 2 particles with sub-micrometer size, as revealed by scanning electron microscopy (SEM) images ( Supplementary Fig. 1 ) [24] . The electrochemical tuning process of the pristine LiCoO 2 in 1:1 volume mix of ethylene carbonate and diethyl carbonate electrolyte (1 M LiPF 6 ) was recorded in Fig. 1b , where we could see the material was charged to 4.3 V (versus Li + /Li) along with a delithiation reaction, equation (2). On the basis of the calculated charge capacity, approximately half of the Li in the LiCoO 2 was extracted, leading to the formation of Li 1− x CoO 2 ( x ≈0.5) [21] , [22] . The OER catalytic activities of LiCoO 2 and De-LiCoO 2 were evaluated by steady-state electrochemistry measurements in a 0.1-M KOH aqueous solution using a typical three-electrode cell setup (see Methods). All the electrochemical measurement data had been corrected with a resistance drop of ~20 Ω. The polarization curve recorded with the LiCoO 2 showed a large onset potential (defined as the potential at an OER current density of 0.1 mA cm −2 ) of ~1.59 V for the OER ( Fig. 2a , black line), beyond which the anodic current rose slowly by applying higher overpotential (ca. a current density of ~2.3 mA cm −2 at ~1.7 V). This poor OER activity of LiCoO 2 was consistent with the data observed previously [25] . In sharp contrast, De-LiCoO 2 showed markedly improved OER activity with a reduced onset potential of ~1.52 V (red line in Fig. 2a ) and fast current increase (ca. ~3.8 mA cm −2 at ~1.6 V). Considering the Tafel slopes of ~50 mV dec −1 for both samples ( Fig. 2b ), the shift in onset potential correlated with over one order of magnitude enhancement of OER activity. The effective surface areas of the samples before and after delithiation were estimated by measuring the capacitance of the double layer (EDLC, electric double layer capacitance) at the solid–liquid interface with cyclic voltammetry ( Supplementary Fig. 2 ) [26] . The EDLC of De-LiCoO 2 electrode was estimated to be ~2,000 μF cm −2 while that of original LiCoO 2 was only ~60 μF cm −2 . These results indicated that, although no obvious pulverization or other morphological changes were observed in De-LiCoO 2 particles comparing SEM images ( Supplementary Fig. 1 ), the electrochemically active sites of De-LiCoO 2 catalyst were much more than that of LiCoO 2 catalyst, which is consistent with the enhanced OER activity in De-LiCoO 2 . 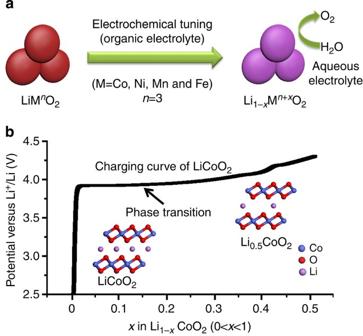Figure 1: Schematic of the electrochemical lithium tuning process. (a) Schematic illustration of the electrochemical tuning process of LiMO2(M=Co, Ni, Mn and Fe), where the oxidation state of M center would be higher after electrochemical tuning in organic electrolyte and suitable for water oxidation in aqueous electrolyte. (b) A typical charging curve of LiCoO2. The crystal structure of the material and the electronic structure of the Co atom are both changed after phase transition, which occurred at the potential of 3.9–4 V versus Li+/Li. Figure 1: Schematic of the electrochemical lithium tuning process. ( a ) Schematic illustration of the electrochemical tuning process of LiMO 2 (M=Co, Ni, Mn and Fe), where the oxidation state of M center would be higher after electrochemical tuning in organic electrolyte and suitable for water oxidation in aqueous electrolyte. ( b ) A typical charging curve of LiCoO 2 . The crystal structure of the material and the electronic structure of the Co atom are both changed after phase transition, which occurred at the potential of 3.9–4 V versus Li + /Li. 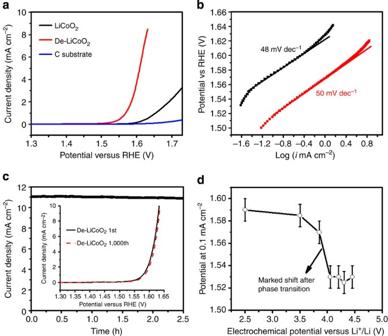Figure 2: OER performance of De-LiCoO2upon delithiation. (a) Polarization curves of LiCoO2and De-LiCoO2. (b) Tafel plots of LiCoO2(black curve) and De-LiCoO2(red curve). (c) 1st and 1,000th polarization curves of De-LiCoO2. (d) Plots of the electrochemical tuning potentials versus required OER potentials of LiCoO2at 0.1 mA cm−2. The error bars of the potentials are defined by calculating the relative deviations for at least five independent measurements. Full size image Figure 2: OER performance of De-LiCoO 2 upon delithiation. ( a ) Polarization curves of LiCoO 2 and De-LiCoO 2 . ( b ) Tafel plots of LiCoO 2 (black curve) and De-LiCoO 2 (red curve). ( c ) 1st and 1,000th polarization curves of De-LiCoO 2 . ( d ) Plots of the electrochemical tuning potentials versus required OER potentials of LiCoO 2 at 0.1 mA cm −2 . The error bars of the potentials are defined by calculating the relative deviations for at least five independent measurements. Full size image The long-term stability of a catalytic electrode is another critical issue to consider for commercial applications. Especially, it is a practical concern for the delithiated sample, as it is produced at a high electrochemical potential. In this case, the polarization curve of De-LiCoO 2 after 1,000 cycles almost overlaid the curve of the first cycle with negligible loss of anodic current, and a stable current of ~10 mA cm −2 was observed for >2 h operating, both indicating a good durability of the catalyst ( Fig. 2c ). We also measured the OER activity of pure carbon black on carbon substrate (blue curve in Fig. 2a ), which showed negligible current density in the potential <1.6 V, indicating that the high anodic current density observed with the De-LiCoO 2 catalyst was dominant for OER rather than oxidation of carbon. In addition, the generated gas was confirmed to be pure O 2 using gas chromatography, which also revealed a Faradaic efficiency similar to that of an IrO 2 benchmark ( Supplementary Fig. 3 ). Structural analysis for the enhanced OER performance The structural and compositional analysis on LiCoO 2 and De-LiCoO 2 may shed light on tracing the source for the improved OER activity. The X-ray diffraction (XRD) pattern of the pristine LiCoO 2 showed good hexagonal ordering and layered characteristics ( Fig. 3a , black line), while a monoclinic phase was found on the De-LiCoO 2 ( Fig. 3a , red line) [21] , [22] . The positions and intensities of the peaks of De-LiCoO 2 matched well with the refined XRD pattern of Li 0.5 CoO 2 (ref. 27 ), and the most obvious change before and after delithiation was the disappearance of the original (003) peak (2 θ ≈19°) and the appearance of a new peak at a lower angle (2 θ ≈18.4°) as shown in Fig. 3b (ref. 21 ), confirming the formation of Li 0.5 CoO 2 in De-LiCoO 2 . The observed broader width and slightly shifted position of the peak located at ~18.4° may suggest that the as-prepared De-LiCoO 2 showed less ordering. Although the valency change of Co could not be clearly resolved by the X-ray photoelectron spectroscopy (XPS) result ( Supplementary Fig. 4 ) similar to previous work [28] , we believe the oxidation state of Co should be higher than 3+ after the electrochemical tuning process according to the XRD results. It should be noted that such an electrochemical tuning of crystal structure and oxidation states of Co center can be realized in organic lithium electrolyte, but it does not take place in 0.1 M KOH aqueous electrolyte. As shown in the XRD data ( Fig. 3c,d ), there is no peak shift in the XRD patterns for LiCoO 2 and De-LiCoO 2 after holding the catalysts at an OER potential (1.8 V versus RHE) for several hours in 0.1 M KOH aqueous electrolyte. Therefore, the new electronic and crystal structure formed by electrochemical tuning in organic lithium electrolyte can be maintained during OER in aqueous electrolyte. These data are consistent with the stability performance of the catalyst. 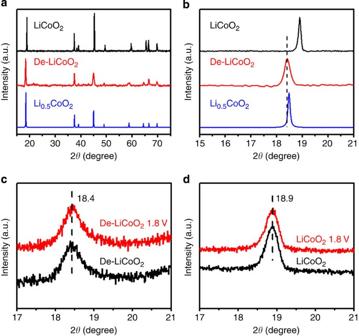Figure 3: Structural analysis of LiCoO2before and after electrochemical tuning. (a) Powder XRD patterns of LiCoO2, De-LiCoO2and Li0.5CoO2(the XRD pattern of Li0.5CoO2was refined by the lattice parameters in ref.22). (b) Localized XRD patterns with the 2θrange from 15–21°. (c) Localized XRD patterns of De-LiCoO2loaded on a current collector before (black line) and after (red line) holding at 1.8 V versus reversible hydrogen electrode (RHE) for >2 h. (d) Localized XRD patterns of LiCoO2loaded on a current collector before (black line) and after (red line) holding at 1.8 V versus RHE for >2 h. Figure 3: Structural analysis of LiCoO 2 before and after electrochemical tuning. ( a ) Powder XRD patterns of LiCoO 2 , De-LiCoO 2 and Li 0.5 CoO 2 (the XRD pattern of Li 0.5 CoO 2 was refined by the lattice parameters in ref. 22 ). ( b ) Localized XRD patterns with the 2 θ range from 15–21°. ( c ) Localized XRD patterns of De-LiCoO 2 loaded on a current collector before (black line) and after (red line) holding at 1.8 V versus reversible hydrogen electrode (RHE) for >2 h. ( d ) Localized XRD patterns of LiCoO 2 loaded on a current collector before (black line) and after (red line) holding at 1.8 V versus RHE for >2 h. Full size image The electrochemical potential of LiCoO 2 can be tuned within a wide range, as shown in Fig. 1b . A key question is whether the different tuning potential in organic electrolyte can change the OER activity. Since the phase transition of LiCoO 2 to Li 0.5 CoO 2 takes place between 3.9 and 4 V, we would expect a large change of OER activity around this transition potential. Figure 2d summarized the required OER potentials for delivering 0.1 mA cm −2 at different tuning potentials of 2.5 (open-circuit potential), 3.5, 3.85, 4.05, 4.2, 4.3 and 4.45 V versus Li + /Li electrode (the detailed polarization curves can be seen in Supplementary Fig. 5 ). It is clearly shown that the samples after tuning potential larger than 4 V show the markedly enhanced OER performance, which comes from the Li 0.5 CoO 2 phase. The Li 0.5 CoO 2 phase possesses a higher activity than the LiCoO 2 phase, which may originate from the change of the electronic structure. Previous reports [28] , [29] , [30] , [31] have shown that the electron charge transfer resulting from Li+ extraction simultaneously involves cobalt and oxygen, which can both be considered to undergo a partial oxidation process, and that more charge is transferred to the oxygen ions than to the metal ions. Therefore, the enhanced OER activity of De-LiCoO 2 may be attributed to the following possible reasons. First, the increased oxidation state of Co in Li 0.5 CoO 2 phase to a valency that is >3+ can enhance the electrophilicity of the adsorbed O, and thus facilitate the reaction of an OH- anion with an adsorbed O atom on the catalytic active sites to form adsorbed −OOH species [17] , [18] , which is considered as the rate-limiting step for OER [9] . Experimentally, the model is also supported by the promotion effect of molecular cobaltate clusters on water oxidation if the Co valency is >3 (ref. 17 ). Second, the Co–O bond becomes more covalent upon the delithiation process, which may also lead to the formation of holes in the hybridized Co 3 d —O 2 p band. This change can also make the material more electrophilic, thus facilitating the adsorption of the hydroxyl group, resulting in enhanced OER activity. Third, it is revealed that LiCoO 2 is a semiconductor, whereas Li 0.5 CoO 2 is metallic [27] , thus the efficient charge transport through conductive support to catalyst surface in metallic De-LiCoO 2 is also likely beneficial to OER activity. Tuning mixed metal oxides for improving OER activity Mixed transition metal oxides usually show superior OER activity compared to either of the parent metal oxides. It was reported that Ni doping in Co oxides could lead to the creation of new active sites with lower activation energy [32] , [33] , and Fe dopants were found to enhance the OER activities of Ni hydroxides or oxides [11] , [34] , [35] , [36] , [37] . Recently, an excellent OER performance was observed on amorphous NiCoFe oxides, which were prepared by a photochemical route [38] , [39] . We were intrigued to find out whether our electrochemical lithium tuning method is generally effective in tuning the electronic structure of mixed transition metal oxides towards even better OER activity. We introduced an additional three transition metals (Ni, Fe and Mn) into the pristine LiCoO 2 structure to form a series of Co-based mixed metal oxides: LiCo 0.5 Ni 0.5 O 2 , LiCo 0.5 Fe 0.5 O 2 , LiCo 0.33 Ni 0.33 Fe 0.33 O 2 and LiCo 0.33 Ni 0.33 Mn 0.33 O 2 . XRD data and further analysis ( Fig. 4a ; Supplementary Fig. 6 ; Supplementary Table 1 ; Supplementary Note 1 ) suggest that mixed phases are found in the samples, which are mainly composed of layered lithium transition metal oxides. As expected, the pristine oxides with mixed transition metals (Ni or Fe) showed slightly improved OER activities compared with pristine LiCoO 2 (see Fig. 4b,c ). After electrochemical tuning to a higher potential of 4.3 V versus Li, the corresponding delithiated mixed oxides (denoted as De-LiCo 0.5 Ni 0.5 O 2 , De-LiCo 0.5 Fe 0.5 O 2 , De-LiCo 0.33 Ni 0.33 Fe 0.33 O 2 and De-LiCo 0.33 Ni 0.33 Mn 0.33 O 2 ) all showed appreciable improvements ( Fig. 4b , solid lines and Supplementary Fig. 7 ). For all the samples, the onset potential decreased by around 30–80 mV after the electrochemical tuning process ( Fig. 4c ). In addition, the delithiated mixed oxides exhibited comparable or improved Tafel slopes, indicating that this tuning process would not induce a negative effect on OER kinetics ( Supplementary Fig. 8 ). Moreover, repeated potential cycling test for 1,000 cycles with the higher bound of the current density of ~10 mA cm −2 ( Fig. 4d ; Supplementary Fig. 9 ) demonstrated the high stability of delithiated samples, thus making these catalysts promising for practical applications. However, the delithiation process may not be applicable to other systems ( Supplementary Fig. 10 ). 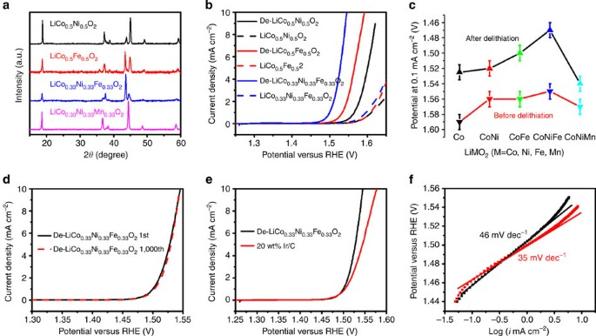Figure 4: OER improvements on other mixed metal oxides by electrochemical tuning. (a) XRD patterns of mixed lithium transition metal oxides. (b) Polarization curves of mixed lithium transition metal oxides before and after delithiation. (c) Onset potentials (potentials required to reach 0.1 mA cm−2) of the various catalysts for OER, the error bars are defined by at least five independent measurements. (d) Cycling stability of De-LiCo0.33Ni0.33Fe0.33O2catalyst. (e) Comparison of polarization curves of De-LiCo0.33Ni0.33Fe0.33O2and 20 wt% Ir/C catalysts. (f) Tafel slopes of De-LiCo0.33Ni0.33Fe0.33O2and 20 wt% Ir/C catalysts. The error bars in panelcare defined by calculating the relative deviations from more than 5 independent experiments. Figure 4: OER improvements on other mixed metal oxides by electrochemical tuning. ( a ) XRD patterns of mixed lithium transition metal oxides. ( b ) Polarization curves of mixed lithium transition metal oxides before and after delithiation. ( c ) Onset potentials (potentials required to reach 0.1 mA cm −2 ) of the various catalysts for OER, the error bars are defined by at least five independent measurements. ( d ) Cycling stability of De-LiCo 0.33 Ni 0.33 Fe 0.33 O 2 catalyst. ( e ) Comparison of polarization curves of De-LiCo 0.33 Ni 0.33 Fe 0.33 O 2 and 20 wt% Ir/C catalysts. ( f ) Tafel slopes of De-LiCo 0.33 Ni 0.33 Fe 0.33 O 2 and 20 wt% Ir/C catalysts. The error bars in panel c are defined by calculating the relative deviations from more than 5 independent experiments. Full size image The parameters to describe the activity of the pristine and delithiated oxides catalysts are summarized in Table 1 . The most efficient OER catalyst identified in our study was the De-LiCo 0.33 Ni 0.33 Fe 0.33 O 2 (the electrochemical tuning process is shown in Supplementary Fig. 11 ), which possessed a small onset potential of ~1.47 V versus RHE and a low Tafel slope of ~35 mV dec −1 ( Fig. 4e,f ). For comparison, a commercial 20 wt% Ir/C catalyst with the same mass loading (~0.1 mg cm −2 ) exhibited a similar onset potential (~1.46 V), but a larger Tafel slope (~46 mV dec −1 ). Accordingly, the OER current density of Ir/C increased slowly with higher overpotential and fell below our De-LiCo 0.33 Ni 0.33 Fe 0.33 O 2 at ~1.5 V. Therefore, De-LiCo 0.33 Ni 0.33 Fe 0.33 O 2 is superior to Ir/C catalyst to drive significant anodic current densities for OER (1–10 mA cm −2 ). Table 1 Summary of OER activities. Full size table In summary, the electrochemical tuning (delithiation) process in organic electrolyte has been demonstrated as an effective route to enhance the OER activity of LiCoO 2 in aqueous solution. This improvement was attributed to the formation of the monoclinic phase of Li 0.5 CoO 2 , which offers a more desirable electronic structure to drive the catalytic reaction. The electrochemical tuning efficacy is shown to be general in many Co-based mixed metal oxides. Particularly, the De-LiCo 0.33 Ni 0.33 Fe 0.33 O 2 exhibited optimal activity, better than the commercial Ir/C catalyst. In the future, we will extend this methodology to a wide range of catalytic materials and study its broader applicability. The work here on Co-based oxides together with previous demonstration of electrochemically tuned MoS 2 for better HER activity have shown the promise of this methodology to improve heterogeneous electrocatalysts, not only for the OER in water, but also for efficient, rechargeable metal-air batteries, regenerative fuel cells and other rechargeable air-based energy storage devices. Synthesis of lithium transition metal oxides The lithium transition metal oxides were synthesized by following procedures in a previous study [24] . In all cases, cotton obtained from a local drug store were soaked in solutions of lithium nitrate (LiNO 3 ) and transition metal nitrate (Co(NO 3 ) 2 , Ni(NO 3 ) 2 , Fe(NO 3 ) 3 and Mn(NO 3 ) 2 ), purchased from Sigma-Aldrich, in de-ionized water with a 1:1 molar ratio. The total salt concentration of 0.33 M was employed. For instance, the solution containing LiNO 3 and Co(NO 3 ) 2 was used to synthesize LiCoO 2 . After soaking for 3 h, the cotton was taken out and then squeezed to remove excessive liquid. The damp cotton was placed in a box furnace and heated in air at a rate of 100 °C per hour to a temperature of 400 °C. After cooling, the resulting material was gently hand grounded and returned to the furnace. It was then heated at the same rate to a final temperature of 850 °C, which was maintained for 4 h. Subsequently, the product was taken from the furnace and cooled in air to room temperature. Electrochemical tuning of lithium transition metal oxides The electrochemical tuning process was operated in a pouch battery cell. The electrodes were prepared by making slurries of 80% active material, 15% conducting carbon black and 5% polyvinylidene difluoride binder in an ethanol solvent. Slurries were doctor-bladed onto aluminium foil and dried in a vacuum oven overnight. Afterwards, electrodes were cut out and put into pouch cells, which were assembled in an argon-filled glove box free of oxygen and water. Lithium metal foil was used as the negative electrode, and a 1-M solution of LiPF 6 in ethylene carbonate and diethyl carbonate electrolyte (EC/DEC) (1:1, from Ferro Corporation) was used as the electrolyte. The separator was polypropylene-based Celgard 2321. The delithiation process was performed by charging the cell to a high potential (ca. 4.3 V versus Li+/Li) after two charge/discharge cycles. Consequently, the delithiated product was taken out and rinsed with ethanol several times. Characterization The size and morphology were carried out using SEM (FEI Nova NanoSEM 450). XPS (SSI SProbe XPS spectrometer with Al(Ka) source) was used to measure the valence of the surface Co atoms. The X-ray powder diffraction patterns were recorded on an X-ray diffractometer (Rigaku D/max 2500) in the range from 15 to 60°. Sample preparation and electrochemical characterization For the preparation of the catalytic electrodes, the catalysts before delithiation were dispersed in ethanol to achieve a catalyst concentration of ~1 mg ml −1 with 5 wt% polyvinylidene difluoride and 15 wt% conducting carbon black. The catalysts after delithiation were directly dispersed in ethanol with the same catalyst concentration. After sonication for 45 min, 100 μl of the catalyst ink was drop-dried onto a 1 cm × 1 cm carbon fibre paper (from Fuel Cell Store, the mass loading was ~0.1 mg cm −2 ). The 20 wt% Ir/C catalyst was purchased from Premetek Co. The measurements were performed in 0.1 M KOH solution using a three-electrode setup, with a Hg/HgO reference electrode and a platinum wire counter electrode. The reference electrode was calibrated in H 2 -saturated electrolyte with respect to an in situ RHE, by using two platinum wires as working and counter electrodes, which yielded the relation E(RHE)=E(Hg/HgO)+0.86 V. The electrode was first cycled ~5 times by cyclic voltammetry until a stable cyclic voltammetry curve was developed before measuring polarization curves. Linear sweep voltammetry (scan rate of 2 mV s −1 ) and AC impedance spectroscopy (at zero overpotential) were recorded by a Biologic VSP potentiostat. Gas chromatography measurement OER catalyses were performed in a gas-tight two-compartment electrochemical cell with 1 M KOH electrolyte. The working electrodes were prepared by drop-drying 0.3 mg De-LiCoO 2 into 1 cm 2 carbon fibre paper and 0.3 mg IrO 2 powder (from Premetek Co.) onto 1 cm 2 Nickel foam. Chronopotientiometry was applied with a constant current density of ~10 mA cm −2 , and N 2 was constantly purged into the anodic compartment with a flow rate of 5 cm 3 min −1 and this compartment was connected to the gas-sampling loop of a gas chromatograph (SRI 8610C). A thermal conductivity detector was used to detect and quantify the oxygen generated. How to cite this article: Lu, Z. et al. Electrochemical tuning of layered lithium transition metal oxides for improvement of oxygen evolution reaction. Nat. Commun. 5:4345 doi: 10.1038/ncomms5345 (2014).